High frequency of telomerase reverse-transcriptase promoter somatic mutations in hepatocellular carcinoma and preneoplastic lesions Somatic mutations activating telomerase reverse-trancriptase promoter were recently identified in several tumour types. Here we identify frequent similar mutations in human hepatocellular carcinomas (59%), cirrhotic preneoplastic macronodules (25%) and hepatocellular adenomas with malignant transformation in hepatocellular carcinomas (44%). In hepatocellular tumours, telomerase reverse-transcripase- and CTNNB1 -activating mutations are significantly associated. Moreover, preliminary data suggest that telomerase reverse-trancriptase promoter mutations can increase the expression of telomerase transcript. In conclusion, telomerase reverse-trancriptase promoter mutation is the earliest recurrent genetic event identified in cirrhotic preneoplastic lesions so far and is also the most frequent genetic alteration in hepatocellular carcinomas, arising from both the cirrhotic or non-cirrhotic liver. Hepatocellular carcinoma (HCC) is a highly heterogeneous disease at the clinical, pathological and molecular levels. More than 80% of HCC develop from a cirrhotic liver after exposure to specific risk factors mainly represented by hepatitis B (HBV) and C viral infections, alcohol intake, obesity and rare genetic diseases [1] . The most frequent genetic alterations identified in HCC are mutations of TP53 and CTNNB1 (15–40%) [2] . Recent studies using whole-exome sequencing have revealed recurrent mutations in new driver genes involved in the chromatin remodelling ( ARID1A and ARID2 ), in the ras/raf/map kinase ( RPS6KA3 ) and the oxidative stress ( NFE2L2 ) pathways [3] , [4] . However, no recurrent somatic mutations were described in cirrhotic macronodules, the principal preneoplastic lesion for HCC development [5] . In 20% of cases, HCCs are developed in the absence of cirrhosis and, rarely, they result from the malignant transformation of hepatocellular adenoma (HCA). Among these benign tumours, adenoma harbouring CTNNB1 -activating mutations are more at risk of malignant transformation leading to the development of an HCC in normal liver [6] . However, CTNNB1 mutations alone are not sufficient for the development of a malignant tumour [7] . Telomerase reverse-trancriptase ( TERT ), coding for telomerase, is also known to be involved in tumorigenesis: rare TERT germline-inactivating mutations are associated to cirrhosis in human [8] , [9] and telomere-deficient mTerc −/− mice are prone to develop HCC but reactivation of telomerase is required for tumour progression [10] , [11] , [12] , [13] . Recently, frequent somatic mutations in the TERT (coding for telomerase reverse transcriptase) promoter have been reported in melanoma [14] , [15] and in several other tumour types [16] . These mutations created a potential binding site for ETS (E-twenty six)/ternary complex factor (TCF) transcription factors and are predicted to increase promoter activity and TERT transcription. In this study, we searched for TERT promoter mutations in a large panel of hepatocellular tumours. We identified TERT promoter mutations as the most frequent somatic genetic alterations in HCC and as the first gene recurrently mutated in cirrhotic preneoplastic lesions. Moreover, TERT promoter mutations were involved at the last step of malignant transformation of HCA. 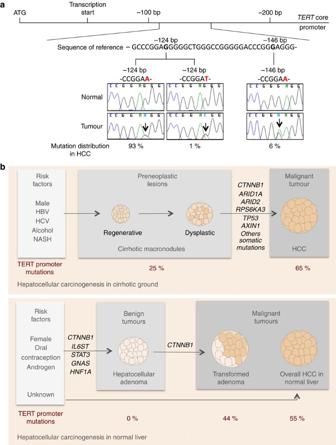Figure 1: Somatic mutations of theTERTpromoter in human liver carcinogenesis. (a) Mutation spectrum of theTERTpromoter in 179 human HCCs: substitution at two hot spots (−124 and −146 bp from the ATG start site, g.1,295,228 and g.1,295,250, respectively) that create a new ETS-/TCF-binding sequences. Distribution (%) of the 179 mutations along theTERTpromoter (59% of all HCCs) is indicated. Mutations are represented on the +strand of DNA. (b)TERTpromoter mutations in the multistep process of liver carcinogenesis. Percentage ofTERTpromoter mutations is reported at each step of liver carcinogenesis. On cirrhosis, 5/20 (25%) cirrhotic macronodules (three with dysplasia and two without dysplasia) and 71/110 (65%) HCCs were mutated forTERT. On normal liver, no mutations of theTERTpromoter (0%) were identified among 60 HCAs; in contrast, 7/16 (48%) of malignant transformation of HCA and 58/106 (55%) of HCCs without signs of malignant transformation from HCA exhibited mutations of theTERTpromoter. Other genes most frequently mutated in HCC and HCA are indicated. TERT promoter mutations in HCCs We sequenced the promoter region of TERT using direct Sanger technique in 305 HCCs related to various risk factors and surgically resected in two French university hospitals ( Table 1 ) [17] . We found recurrent somatic mutations in 179 HCCs (59%) at the two hot spots previously described ( Supplementary Table S1 ) [14] , [15] , [16] . Among 24 hepatocellular cell lines tested, TERT promoter mutations were identified in 15 cases (63%; Supplementary Table S2 ). The most frequent mutations were located at −124 bp from the ATG start site, they consist in G to A (−124G>A, 166 cases, 93%) or G to T (−124G>T, two cases, 1%) substitutions ( Fig. 1a and Supplementary Table S1 ). The second hot spot was situated at −146 bp from the ATG and characterized by G to A substitutions (−146G>A, 11 cases, 6%; Fig. 1a and Supplementary Table S1 ). The mutations create a typical ETS/TCF-binding sequence, as previously described [14] , [15] , [18] . We confirmed that all mutations were somatic and mutations at the two hot spots were mutually exclusive. In contrast to melanoma, we did not found any tandem GG>AA mutations, a hallmark of ultraviolet-induced mutagenesis. In addition, mutations at −146 bp were significantly less frequent in HCC (6% of all TERT promoter mutations) than that in melanoma (46% of all TERT promoter mutations, P <0.0001, Fisher’s exact test) [14] , [15] . Together, these data suggest that the somatic mutations in the TERT promoter are the most frequent genetic alterations in human HCC ( Fig. 1b ). Table 1 Characteristics of the patients according to presence or absence of TERT promoter mutations ( n =305). Full size table Figure 1: Somatic mutations of the TERT promoter in human liver carcinogenesis. ( a ) Mutation spectrum of the TERT promoter in 179 human HCCs: substitution at two hot spots (−124 and −146 bp from the ATG start site, g.1,295,228 and g.1,295,250, respectively) that create a new ETS-/TCF-binding sequences. Distribution (%) of the 179 mutations along the TERT promoter (59% of all HCCs) is indicated. Mutations are represented on the +strand of DNA. ( b ) TERT promoter mutations in the multistep process of liver carcinogenesis. Percentage of TERT promoter mutations is reported at each step of liver carcinogenesis. On cirrhosis, 5/20 (25%) cirrhotic macronodules (three with dysplasia and two without dysplasia) and 71/110 (65%) HCCs were mutated for TERT . On normal liver, no mutations of the TERT promoter (0%) were identified among 60 HCAs; in contrast, 7/16 (48%) of malignant transformation of HCA and 58/106 (55%) of HCCs without signs of malignant transformation from HCA exhibited mutations of the TERT promoter. Other genes most frequently mutated in HCC and HCA are indicated. Full size image Among the 305 screened HCCs, we observed that TERT promoter mutations were more frequent in men ( P =0.001, χ 2 -test), in patients with low serum levels of alpha-fetoprotein ( P =0.01, χ 2 -test), in small tumours of <5 cm ( P =0.01, χ 2 -test), non-related to HBV ( P <0.0001, χ 2 -test) and mutated for CTNNB1 ( P <0.0001, χ 2 -test, Fig. 1b and Table 1 ). Interestingly, TERT expression assessed by quantitative reverse transcription (RT)–PCR was increased in HCC harbouring TERT promoter mutations compared with normal liver, cirrhosis and HCA ( P =0.0007, Mann–Whitney test, Fig. 2a ). Within the malignant liver tumours, TERT expression was increased (fold change tumour/normal liver>10) in almost all HCCs exhibiting TERT promoter mutation (92%), whereas HCCs non-mutated for TERT promoter overexpressed less frequently TERT messenger RNA (80%; P =0.007, Fisher’s exact test). 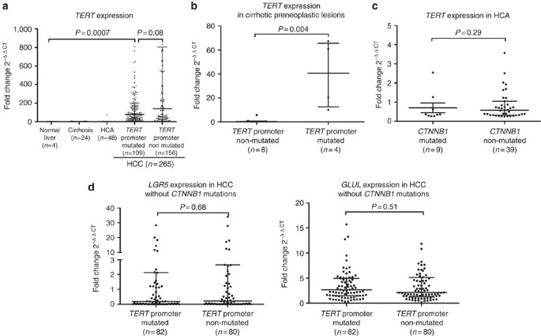Figure 2:TERTtranscript expression according to mutation status of theTERTpromoter. (a)TERTmessenger RNA (mRNA) is not expressed in 4 normal livers, 24 cirrhosis and 48 HCAs, whereas it is overexpressed in 156 HCCs mutated and 109 HCCs not mutated for theTERTpromoter. (b)TERTtranscript was overexpressed in all mutated cirrhotic macronodules (n=4) when compared with non-mutated macronodules (n=8). (c)TERTmRNA was not overexpressed in HCA withCTNNB1mutations (n=9) compared with HCA without CTNNB1 mutations (n=39). (d) β-catenin target genes (GLULandLGR5) were not overexpressed in HCC harbouringTERTpromoter mutations withoutCTNNB1mutations (n=82) compared with HCC lacking bothTERTpromoter andCTNNB1mutations (n=80).TERT, GLUL and LGR5mRNA levels were measured using quantitative RT–PCR. All the results were normalized with the mean of normal liver tissues (see Methods section). Results were reported in median with interquartile range and compared using non-parametric Mann–Whitney test. Differences were considered significant when theP-value was <0.05. Figure 2: TERT transcript expression according to mutation status of the TERT promoter. ( a ) TERT messenger RNA (mRNA) is not expressed in 4 normal livers, 24 cirrhosis and 48 HCAs, whereas it is overexpressed in 156 HCCs mutated and 109 HCCs not mutated for the TERT promoter. ( b ) TERT transcript was overexpressed in all mutated cirrhotic macronodules ( n =4) when compared with non-mutated macronodules ( n =8). ( c ) TERT mRNA was not overexpressed in HCA with CTNNB1 mutations ( n =9) compared with HCA without CTNNB1 mutations ( n =39). ( d ) β-catenin target genes ( GLUL and LGR5 ) were not overexpressed in HCC harbouring TERT promoter mutations without CTNNB1 mutations ( n =82) compared with HCC lacking both TERT promoter and CTNNB1 mutations ( n =80). TERT, GLUL and LGR5 mRNA levels were measured using quantitative RT–PCR. All the results were normalized with the mean of normal liver tissues (see Methods section). Results were reported in median with interquartile range and compared using non-parametric Mann–Whitney test. Differences were considered significant when the P -value was <0.05. Full size image TERT promoter mutations in cirrhotic preneoplastic lesions To search for early genetic events in preneoplastic lesions, we screened for TERT promoter mutations in 69 cirrhotic tissues and 20 cirrhotic macronodules with or without dysplasia (13 and 7 cases, respectively, Supplementary Table S3 ). We identified a somatic TERT promoter mutation in five macronodules (25%) with (three cases) or without (two cases) dysplasia, whereas none of the cirrhotic tissues were mutated. Accordingly, we showed that TERT promoter mutations in macronodules were associated with an increased transcription of telomerase, whereas TERT was not overexpressed in cirrhosis and non-mutated macronodules ( P =0.004, Mann–Whitney test, Fig. 2a and b ). Moreover, we screened 15 of these cirrhotic macronodules for mutations in 10 genes that are the most frequently mutated in HCC ( CTNNB1 , ARID1A , ARID2 , RPS6KA3 , NFE2L2 , TP53 , KRAS , PIK3CA , AXIN1 and CDKN2A ), and no somatic variants were identified. Altogether, these results identified TERT promoter mutation as the first recurrent genetic alteration in cirrhotic preneoplastic macronodules. In addition, it revealed TERT as the earliest genomic event currently identified in the multistep process of liver carcinogenesis on cirrhosis ( Fig. 1b ). TERT promoter mutations in malignant transformation of HCA Next, we screened 60 typical HCAs of various molecular subclasses without signs of malignant transformation, and no mutations were identified in TERT promoter ( Supplementary Table S4 ). In contrast, in a series of 16 HCAs with malignant transformation (‘nodule in nodule’ or HCA with HCC foci) we found TERT promoter mutations in seven cases (44%), all associated with a CTNNB1 -activating mutation ( Supplementary Table S5 ). These data show that somatic mutations of the TERT promoter are not required for clonal benign hepatocellular tumorigenesis but they are critical for malignant transformation of HCA in addition to CTNNB1 mutations ( Fig. 1b ). Finally, in other HCC developed in normal liver, TERT promoter mutations are frequent (55%, Fig. 1b ) and they are also significantly associated with CTNNB1 -activating mutations. Interestingly, β-catenin were previously identified as an activator of TERT in embryonic stem cell and in intestinal hyperplasia developed in mice [19] . Here in HCA mutated for CTNNB1 and without TERT promoter mutation, we did not observe an increased transcription of TERT ( Fig. 2c ). In another study, Park et al. [20] identified telomerase as an activator of the Wnt/β-catenin signalling in cooperation with BRG1, a SWI/SNF-related chromatin remodelling protein [21] . In the present study, in HCC demonstrating a TERT promoter mutation and without CTNNB1 mutation we did not observe a significant increase of expression in the β-catenin target genes ( GLUL and LGR5 ) compared with HCC without TERT and CTNNB1 promoter mutations ( Fig. 2d ). These results suggested that in tumour hepatocytes, β-catenin may not control directly TERT transcription and vice versa . In this study, we identified TERT promoter mutations in 59% of HCC and in 25% of cirrhotic macronodules with or without dysplasia. It is the most frequent somatic genetic alterations in HCC and also the first recurrent gene somatically mutated in preneoplastic cirrhotic lesions. In addition, classical driver genes the most frequently mutated in liver carcinogenesis ( CTNNB1 , ARID1A , ARID2 , RPS6KA3 , NFE2L2 , TP53 , KRAS , PIK3CA , AXIN1 , CDKN2A ) [3] were identified only in HCC and not in dysplastic macronodules. This finding suggests that mutations of the TERT promoter are the earliest genetic events described so far in the multistep process of carcinogenesis on cirrhosis. In contrast, in benign tumorigenesis in the normal liver, we have previously described several driver genes recurrently mutated including HNF1A , CTNNB1 , IL6ST , GNAS or STAT3 (ref. 6 ). Moreover, HCA harbouring a CTNNB1 mutation have a higher risk of malignant transformation [7] , [22] . We found TERT promoter mutations in malignant transformation of HCA but not in classical HCA without dysplasia. It underlines that TERT promoter mutations are involved at the last step of malignant transformation in association with CTNNB1 mutations. This association between TERT promoter and CTNNB1 mutations was also found in HCC. Altogether, these data suggested that TERT promoter mutations and activation of the Wnt/β-catenin pathway could cooperate to promote malignant transformation. Previous studies have shown in vitro and in the mice model that TERT could regulate CTNNB1 expression and conversely that β-catenin could bind to TERT promoter and participate to control TERT expression [19] , [20] , [21] . In our study, we showed that CTNNB1 -activating mutations alone did not increase TERT transcription in HCA. In addition, HCC with TERT promoter mutations without CTNNB1 mutations did not exhibit a Wnt/β-catenin activation. Consequently, we did not find a direct transcriptional relationship between TERT and Wnt/β-catenin pathway in benign and malignant liver tumours. However, the limited numbers of cases and the different histological subtypes (HCA and HCC) analysed restrain this conclusion, and the role of TERT and CTNNB1 mutations in tumorigenesis remains to be functionally investigated [15] , [16] . As the functional consequences of TERT promoter mutations on transcription are still unclear, we have also investigated the link between TERT promoter mutation and TERT transcription in liver tissues. We showed an increase in the transcription of TERT in cirrhotic macronodules carrying TERT mutations compared with macronodules without mutations that will require additional validation in a larger series of samples. Interestingly, both HCC with TERT promoter mutations and HCC without mutations exhibited an increase in TERT transcription. It suggests that telomerase reactivation is a hallmark of HCC possibly explained by TERT promoter mutations but also by alternative mechanisms [23] , [24] . In particular, the lower rate of TERT promoter mutations in HBV-related HCC could be explained by the frequent insertion of HBV DNA in the TERT promoter known to induce telomerase transcription [25] , [26] . In conclusion, TERT promoter mutations are the most frequent somatic genetic alterations in human HCC arising both from cirrhosis and the normal liver. They are early major events in tumorigenesis occurring at preneoplastic stages in cirrhosis and in malignant transformation of HCA in association with WNT/β-catenin pathway activation. Selection of patients This study was approved by our local institutional review board committee (CCPRB Paris, St Louis, 1997 and 2004). All patients gave their informed consent according to the French law [17] . Tumours samples were frozen following the liver resection for tumour in French University hospitals. We included a total of 401 liver samples including 305 HCCs, 60 typical HCAs, 16 HCAs with signs of malignant transformation and 20 cirrhotic preneoplastic nodules. Patients and tumours features are detailed in Table 1 for HCC, Supplementary Table S3 for cirrhotic preneoplastic lesions, Supplementary Table S4 for HCA without malignant transformation and in Supplementary Table S5 for HCA with malignant transformation. In addition, we studied a series of 24 hepatocellular cell lines ( Supplementary Table S2 ). We also included a series of 69 cirrhotic tissues of various aetiologies (alcohol n =19, HBV n =14, HCV n =31, haemochromatosis n =3, other aetiologies n =2). Tumour and non-tumour liver samples were frozen immediately after surgery and conserved at −80 °C. Tissue samples from the frozen counterpart were also fixed in 10% formaldehyde, paraffin-embedded and stained with haematoxylin and eosin and Masson’s trichrome. The diagnosis of liver tumours was based on established histological criteria [27] , [28] by expert pathologists (JC and PBS). Sequencing After amplification using additives dimethylsulphoxide 5%/glycerol 5% (annealing 62 °C), the TERT promoter was sequenced by Sanger’s direct sequencing using forward 5′-(CAGCGCTGCCTGAAACTC)-3′ and reverse 5′-(GTCCTGCCCCTTCACCTT)-3′ primers [15] . All mutations were confirmed by sequencing a second independent amplification product on both strands and the somatic or germline status was assessed by sequencing the corresponding non-tumour liver. All HCAs were screened for CTNNB1 , IL6ST , HNF1A , GNAS and STAT3 mutations ( Supplementary Table S6 ) and results were already reported [7] , [29] , [30] , [31] . All HCCs were screened for CTNNB1 and TP53 mutations and results were already reported [32] . Preneoplastic cirrhotic lesions (regenerative macronodules, low-grade dysplatic macronodules and high-grade dysplastic macronodules) were screened for CTNNB1 , ARID1A , ARID2 , RPS6KA3 , NFE2L2 , TP53 , KRAS , PIK3CA , AXIN1 , CDKN2A mutations ( Supplementary Table S6 ) [3] . Quantitative RT–PCR Expression was assessed by quantitative RT–PCR in duplicate using TaqMan (Applied Biosystems) gene expression assay (TERT Hs00972656_m1, GLUL Hs00374213_m1 and LGR5 Hs00173664_m1). The relative amount of RNA was calculated with the 2-delta delta CT method [32] . Gene expression was normalized with the RNA ribosomal 18S, and the level of expression of the tumour sample was compared with the mean level of the gene expression in normal liver tissues and expressed as an n -fold ratio. Statistical analysis Continuous/quantitative data were compared using the Kruskall–Wallis or Mann–Whitney test. Dichotomous data, along with independence and measures of association, were analysed using the χ 2 -test (group size of >5) with Yates’ continuity correction or Fisher’s exact test (group size of ≤5) except for multiple variable comparisons ( χ 2 -test two sided). P -values were adjusted for multiple comparisons using Monte–Carlo resampling. All reported P -values were two tailed, and differences were considered significant when the P -value was <0.05. Statistical analysis was performed using the R software. How to cite this article: Nault, J. C. et al. High frequency of telomerase reverse-transcriptase promoter somatic mutations in hepatocellular carcinoma and preneoplastic lesions. Nat. Commun. 4:2218 doi: 10.1038/ncomms3218 (2018).